The use of silk-based devices for fracture fixation Metallic fixation systems are currently the gold standard for fracture fixation but have problems including stress shielding, palpability and temperature sensitivity. Recently, resorbable systems have gained interest because they avoid removal and may improve bone remodelling due to the lack of stress shielding. However, their use is limited to paediatric craniofacial procedures mainly due to the laborious implantation requirements. Here we prepare and characterize a new family of resorbable screws prepared from silk fibroin for craniofacial fracture repair. In vivo assessment in rat femurs shows the screws to be self-tapping, remain fixed in the bone for 4 and 8 weeks, exhibit biocompatibility and promote bone remodelling. The silk-based devices compare favourably with current poly-lactic- co -glycolic acid fixation systems, however, silk-based devices offer numerous advantages including ease of implantation, conformal fit to the repair site, sterilization by autoclaving and minimal inflammatory response. The advent of reliable resorbable device systems has altered the landscape for conditions requiring osseous fixation [1] . Approximately three million facial injuries occur annually, and the American Society of Plastic Surgeons reported over 200,000 craniomaxillofacial surgical procedures in 2012, which is a 164% increase from 2000 and a 7% increase from 2011 (ref. 2) [2] . High-impact fractures have a mortality rate as high as 12% [3] . Currently, metal alloys are the gold standard for fracture-fixation devices, despite their numerous disadvantages, which include extreme stiffness causing stress shielding of the underlying bone, potentially poor wound healing and plate exposure, infection and in some cases the need for removal of metallic implants after fracture healing is complete as in the lower extremity [4] , [5] . Stress shielding may result in a reduction of the density of bone affecting bone remodelling and healing and impacting the mixed dentition when used for paediatric mandible fractures. Metal devices used in paediatric patients may also result in implant migration inciting an inflammatory response in the dura and brain tissue [5] . In addition, metal is incapable of degrading in vivo , may corrode in the body causing pain and inflammation, can create temperature sensitivity and tactile sensation resulting in discomfort for the patient, and can produce problems with visibility [5] , [6] , [7] , [8] , [9] . Recently, the use of resorbable plates and screws composed of poly- L -lactic acid, polyglycolic acid (PGA) and poly-lactic- co -glycolic acid (PLGA) in fracture fixation has reduced the need for hardware removal and resulted in improved bone remodelling after injury by permitting a gradual transfer of stress to the healing bone. These potential benefits have been supported by reports demonstrating favourable results in treating fractures with these resorbable systems [4] , [10] , [11] , [12] , [13] , [14] , [15] . However, conventional resorbable materials are associated with inflammatory reaction, can generate sterile sinus formation, result in incomplete remodelling of the bone and exhibit improper dynamics between device strength retention and wound healing [11] , [12] , [16] . They are primarily limited to specific applications such as paediatric craniofacial reconstruction [10] , fixation of metacarpal fractures [13] , [14] , [15] and long-term soft-tissue moudling [17] due to their lower strength and stiffness. In addition, the fragility of conventional resorbable plates and screws requires careful pre-tapping of the screw hole and insertion while the plates need to be pre-shaped to the exact curvature of the fracture location [14] . Thus, new options for resorbable devices that overcome these limitations would impact surgical practice and expand the use of such devices in a broader range of fixation needs. In the present study, we assess silk-based screws in vitro and in vivo for fixation devices. Silk plates were prepared from the same material and explored from a manufacturing and implantation standpoint and showed feasibility for internal fixation but were not assessed in functional models. Silk is selected due to its robust mechanical features, biocompatibility and FDA-approved (Allergan Medical, Inc.) uses in medical devices. It is degradable in vivo with controllable rates from days to years and has the capability of being functionalized with bioactive compounds [18] , [19] , [20] , [21] , [22] , [23] , [24] . Moreover, silk materials maintain structural stability to >170 °C, are stable at extremes of pH and can be autoclaved for sterilization, all features that enhance potential utility in new medical devices when added to the mechanical features and biocompatibility [25] , [26] . The current study proposes silk screws that are self-tapping, remain fixed in the bone for 4 and 8 weeks, exhibit biocompatibility and promote bone remodelling. The properties of these new silk-based devices compare favourably with those of current PLGA resorbable fixation systems, however, the advantages of the silk systems include an easier implantation technique, conformal fit to the repair site, autoclave sterilization and minimal inflammatory response. Manufacturing and feasibility of silk screws and plates Using a solvent-based process ( Fig. 1 , see Methods), silk blanks were moulded to an average length of 2.5 cm and a diameter of 0.40 cm after drying ( Fig. 2a ). The blanks were then machined into screws (1–72 machine screws, English designation) ( Fig. 2c ) which was chosen as the maximum screw size that could be safely implanted into a rat femur. The major diameter of the screws used for in vitro and in vivo testing was ~1.70 mm. For shear and in vitro enzymatic degradation testing, simple cylindrical pins with a diameter of ~1.50 mm were made to simplify testing and analysis. Silk plates were moulded and machined into samples of various thicknesses and shapes. Once dry, the plates were malleable on hydration and could be formed in situ to fit a patients’ unique anatomy. This is shown in Fig. 2e , where a full skull model’s (Sawbones, USA) orbital fracture was fixed with a 4-hole 100% silk screw and plate system. Fixation was achieved by hydrating the plate with water to allow shaping, pre-drilling holes into the bone using the plate as a guide and inserting the screws without pre-tapping of the hole. While an in vivo fracture fixation was not explored in this study, this preliminary trial exhibits the potential for fracture fixation with silk-based devices. Screws were also implanted into rat femurs and did not require pre-tapping of the bone. 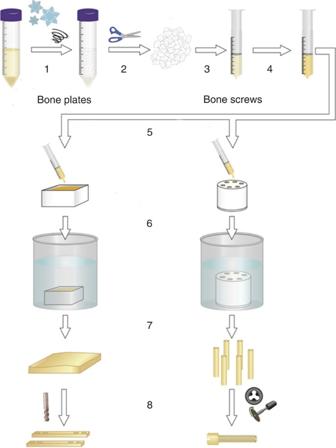Figure 1: Processing diagram of the silk screws and plates. (1) Fill test tube with silk solution then freeze and lyophilize. (2) Use scissors or a blender to cut lyophilized silk into small pieces. (3) Combine pieces with 1,1,1,3,3,3 hexafluoro-2-propanol (HFIP) in a syringe. (4) Dissolve silk in HFIP. (5) Inject dissolved silk into bone plate or screw blank moulds. (6) Place moulds in methanol for 3–4 days to induce β-sheet conversion. (7) Remove and allow to dry (fume hood for 1 week then 60 °C oven for 5 days), then autoclave for stability. (8) Machine using a mill, lathe or die to obtain desired geometry. Figure 1: Processing diagram of the silk screws and plates. (1) Fill test tube with silk solution then freeze and lyophilize. (2) Use scissors or a blender to cut lyophilized silk into small pieces. (3) Combine pieces with 1,1,1,3,3,3 hexafluoro-2-propanol (HFIP) in a syringe. (4) Dissolve silk in HFIP. (5) Inject dissolved silk into bone plate or screw blank moulds. (6) Place moulds in methanol for 3–4 days to induce β-sheet conversion. (7) Remove and allow to dry (fume hood for 1 week then 60 °C oven for 5 days), then autoclave for stability. (8) Machine using a mill, lathe or die to obtain desired geometry. 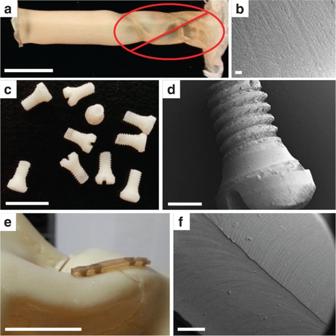Figure 2: General images of the silk devices. (a) Silk blanks prior to machining (scale=6 mm). The left portion of the blank is considered uniform and used for machining while the right portion was discarded due to bubbles and formation of weld lines. (b) SEM image of the surface of silk material after being turned on a lathe (scale=100 μm). (c) Pure silk screws turned on a lathe and then with a 1–72 (English designation) thread-cutting die (scale=6 mm). The major diameter of the screws was ~1.70 mm. (d) SEM image of 1–72 silk screw (scale=1 mm). (e) Combination of silk screws and plates on model skull orbital bone to show fixation potential (scale=25 mm). (f) SEM image of milled surface of silk plate (scale=1 mm). Full size image Figure 2: General images of the silk devices. ( a ) Silk blanks prior to machining (scale=6 mm). The left portion of the blank is considered uniform and used for machining while the right portion was discarded due to bubbles and formation of weld lines. ( b ) SEM image of the surface of silk material after being turned on a lathe (scale=100 μm). ( c ) Pure silk screws turned on a lathe and then with a 1–72 (English designation) thread-cutting die (scale=6 mm). The major diameter of the screws was ~1.70 mm. ( d ) SEM image of 1–72 silk screw (scale=1 mm). ( e ) Combination of silk screws and plates on model skull orbital bone to show fixation potential (scale=25 mm). ( f ) SEM image of milled surface of silk plate (scale=1 mm). Full size image Due to the viscosity of the high-concentration silk solutions, the moudling of silk screw blanks was challenging; the high viscosity did not permit uniform flow and settling of solution into the moulds, resulting in weld lines where different flows met ( Fig. 2a , red circle). Because 1,1,1,3,3,3 hexafluoro-2-propanol (HFIP) is volatile and evaporates quickly, the moulds could not be left in ambient conditions for extended periods of time to allow bubbles to migrate out of the solution. Therefore, it was necessary to place the moulds in methanol within minutes after filling, which prevented the air bubbles from escaping or the solution from completely settling. As a result, half of the blank could be used for machining while the other half was discarded due to non-cylindrical geometry or the presence of bubbles. As indicated in Fig. 2a , it is clear which part of the blank was uniform and which was not. If there was a bubble in the visually uniform portion, the blank would typically break during machining due to mechanical instability. This should not be a problem for making larger screws, as the sizes of the moulds can be increased to increase the amount of usable material for machining without added risk for non-uniformity. Using the uniform portion of the blanks, silk screws were manufactured using standard machining practices. The pure silk blanks were mounted in a lathe, turned down to the desired major diameter and threads were cut using a die. Structure and morphology Fourier transform infrared spectroscopy showed significant β-sheet crystalline fractions in the screw blanks. These fractions define the mechanical properties of silk, thus making it important to have high β-sheet content [27] . As shown in Fig. 3 and Table 1 , the spectra exhibited a distinct peak at 1,621 cm −1 , which is characteristic of β-sheet-rich silk materials, and deconvolution showed a β-sheet content of 51.2±1.45% ( n =6) in the silk screws. Scanning electron microscope (SEM) images showed a smooth surface finish ( Fig. 2b,f ) after machining with the lathe or mill, respectively, and the ability to make reproducible geometries. The screw threads ( Fig. 2d ), while slightly rougher than the machined surfaces, were geometrically reproducible between and within different batches of silk and the increased roughness did not exhibit any deleterious reactions in vivo . The surface roughness could be attributed to the detached silk material that was not properly removed from the screw threads or due to the inconsistency of cutting threads by hand. 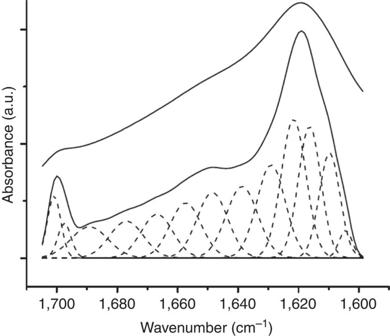Figure 3: FTIR spectroscopy of the silk material. Measurements represent the average of 64 scans taken at a resolution of 4 cm−1(n=6). Peaks at 1,621 cm−1indicate β-sheet conformation while peaks at 1,640 cm−1indicate random coil conformation. FTIR, Fourier transform infrared spectroscopy. Figure 3: FTIR spectroscopy of the silk material. Measurements represent the average of 64 scans taken at a resolution of 4 cm −1 ( n =6). Peaks at 1,621 cm −1 indicate β-sheet conformation while peaks at 1,640 cm −1 indicate random coil conformation. FTIR, Fourier transform infrared spectroscopy. Full size image Table 1 Quantitation of the spectra using deconvolution. Full size table Swelling properties The swelling ratio and water uptake (%) were determined for the silk screws in vitro . The screws had a swell ratio of 0.22±0.03 and a water uptake of 17.9±1.99% ( n =6) after 72 h of hydration in PBS buffer, indicating that this silk format absorbs a significant amount of water. There were no significant differences in weight of the samples between 24, 48 and 72 h ( P >0.05) using a repeated measures ANOVA with Tukey’s multiple comparison test, but to be completely sure the values at 72 h of hydration were used as the ‘equilibrium’ values. The swelling properties of the screws were also assessed in vivo after 4 weeks in the subcutaneous space of rats. The screws yielded a swell ratio of 0.24±0.04 and a water uptake of 19.4±2.45% ( n =12). One-tailed unpaired t -tests for both the swell ratio ( P >0.09) and the water uptake ( P >0.11) of the silk screws in vitro versus in vivo showed there were no significant differences between the samples, signifying that the silk material swells comparably in vitro as in vivo . As described below, the mechanical properties decrease significantly when hydrated. Thus, the swelling timeline was characterized to determine how quickly the material absorbs fluid. This is important with regard to implantation because if the material swells too quickly, resulting in a reduction in mechanical strength, the surgeon may not be able to implant the screws. Samples ( n =6) were placed in 37 °C PBS for various amounts of time (0 min, 1 min, 2 min, 4 min, 8 min, 15 min, 30 min, 60 min, 2 h, 4 h, 24 h, 48 h and 72 h) and observed for changes in weight and diameter to signify fluid uptake and swelling. 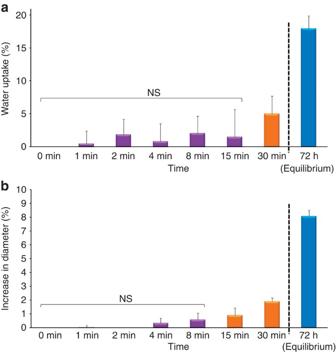Figure 4:In vitroswelling properties. (a) Swelling timeline of the average of six samples with error bars (s.d.) of the water uptake (%) versus time (min). The silk material did not gain a significant amount of weight until after 15 min of incubation in PBS (P>0.05 using Dunnett’s multiple comparison test). The blue bar indicates the water uptake (%) at equilibrium (72 h). (b) Swelling timeline of the average of six samples with error bars (s.d.) showing increase in diameter (%) versus time (min). The silk material did not change diameter significantly until after 8 min of incubation in PBS (P>0.05 using Dunnett’s multiple comparison test). The blue bar indicates the increase in diameter (%) at equilibrium (72 h). Figure 4a shows the water uptake (%) versus time for the first 30 min of testing. A repeated measures ANOVA with Dunnett’s multiple comparison test was performed and showed that samples did not gain a significant amount of weight due to hydration between 0 and 15 min ( P >0.05). After 30 min, the difference in weight was considered significant ( P <0.05). Figure 4b shows the increase in diameter (%) versus time for the first 30 min of testing. For changes in diameter, there were no significant changes between 0 and 8 min ( P >0.05). After 15 min, the change in diameter was considered significant ( P <0.05). We conclude that at least until 8 min, the material does not absorb a significant amount of fluid even if it does come into contact with surrounding tissue or bodily fluids. This time frame is sufficient for the surgeon to implant the screw without concern for hydration and weakening or swelling of the material. Furthermore, the hydration rate will most likely be faster in the in vitro model where the material is in a 100% aqueous environment as compared with brief contact with bodily fluids during a surgery. Figure 4: In vitro swelling properties. ( a ) Swelling timeline of the average of six samples with error bars (s.d.) of the water uptake (%) versus time (min). The silk material did not gain a significant amount of weight until after 15 min of incubation in PBS ( P >0.05 using Dunnett’s multiple comparison test). The blue bar indicates the water uptake (%) at equilibrium (72 h). ( b ) Swelling timeline of the average of six samples with error bars (s.d.) showing increase in diameter (%) versus time (min). The silk material did not change diameter significantly until after 8 min of incubation in PBS ( P >0.05 using Dunnett’s multiple comparison test). The blue bar indicates the increase in diameter (%) at equilibrium (72 h). Full size image Mechanical properties Shear forces are one of the most prominent forces experienced in osseous-fixation devices. Silk pins with a diameter of 1.50 mm, not screws, were used to determine the maximum shear stress, as the simplified geometry allows more straightforward testing and analysis. The pins were tested in shear in dry conditions. The silk pins achieved a maximum shear stress of 90.0±11.8 MPa ( n =8). The pure silk pins were consistent in terms of mechanical properties during dry double lap shear testing and achieved a comparable maximum shear stress to PLGA ( Table 2 ). PLGA screws composed of 82:18 or 80:20 PLA:PGA, commonly used in craniomaxillofacial surgeries, achieve a maximum shear stress of roughly 100 MPa [28] , [29] . Further, improvements to the silk material can be made with the addition of silk micro-fibres or silk micro-particles that have been shown to enhance mechanical properties [30] , [31] . However, the limitation of the current silk format is the hydrated mechanical strength, which is significantly decreased when compared with the dry samples. In the hydrated condition, the pins achieved a maximum shear stress of 19.3±0.51 MPa ( n =6), which was significantly different at the P <0.01 level, using an unpaired t -test with Welch’s correction to account for differences in standard deviations of the dry and hydrated samples. Table 2 Mechanical property comparison table of relevant materials. Full size table Pull-out forces are another common load experienced by bone screws. Silk screws (1–72 designation, 1.70 mm major diameter) were assessed in vitro and in vivo for the pull-out strength ( N ) or the maximum load before failure ( Fig. 5 ). For in vitro testing, the screws were fixed in polyurethane artificial bone blocks, a metallic plate was attached to the screw head and the fixture was extended in the tensile direction until failure. There were two observed failure modes of the screws. First, the screw would pull completely out of the bone with minimal visible damage to the screw. Second, the screw would fracture mid-shaft leaving the bottom of the screw still fixed in the bone. In dry conditions, the screws achieved a maximum load of 80.7±9.38N ( n =6). All six samples pulled completely out of the bone block with minimal visible damage to the screw, implying that the failure was in the polyurethane artificial bone. In hydrated conditions, the screws had a maximum load of 29.0±5.71N ( n =6). Four of the six samples broke along the shank of the screw while two samples pulled completely out of the bone block signifying that the failure was mostly due to the silk material. For in vivo testing, screws were implanted and animals killed after 4 and 8 week time points. Samples were immediately excised with surrounding tissue, bone and screw intact and frozen until testing to minimize tissue degradation and dehydration effects. The samples were thawed and the tissue removed immediately prior to testing to ensure a hydration state similar to in vivo conditions. After 4 weeks in vivo , the screws had a maximum pull-out load of 22.4±5.21N ( n =6). Four of the six samples pulled completely out of the bone while two samples broke along the shank of the screw. After 8 weeks in vivo , the screws achieved a maximum load of 23.3±5.49N ( n =6). Four of the six samples broke along the shank of the screw while two samples pulled completely out of the bone. While not quantifiable or statistically significant, the fact that four of the six 8 week in vivo samples broke along the screw shank, as compared with two out of six 4 week in vivo samples, suggests that there may be more bone ingrowth after 8 weeks. An increased number of samples at longer time points need to be examined to fully quantify the relationship between implant residing time, bone integration and mechanical properties. 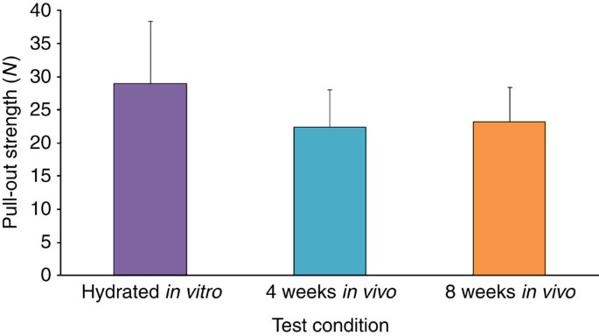Figure 5: Pull-out strength summary. The figure compares hydratedin vitro, 4 weekin vivoand 8 weekin vivodata showing the average of six samples with error bars (s.d). No differences between groups are considered significant withP>0.05 using one-tailed ANOVA with Tukey’s multiple comparison test. Figure 5: Pull-out strength summary. The figure compares hydrated in vitro , 4 week in vivo and 8 week in vivo data showing the average of six samples with error bars (s.d). No differences between groups are considered significant with P >0.05 using one-tailed ANOVA with Tukey’s multiple comparison test. Full size image There are many factors that influence the in vivo pull-out strength tests’ results, such as pilot hole size and depth of insertion that are much harder to control as compared with in vitro models. A one-tailed ANOVA with Tukey’s multiple comparison test was performed and showed no significant differences between hydrated in vitro samples, 4 week and 8 week in vivo samples, signifying that the hydrated in vitro test is a good model for pull-out strength testing. All samples were considered significant as compared with the dry in vitro pull-out strength ( P <0.05). Enzymatic degradation In vitro degradation was observed in the silk samples incubated in 5 U ml −1 of protease XIV at 1, 4 and 8 week time points ( n =3). The samples were 1.50 mm cylindrical geometries of similar sizes to the shanks of silk screws (1.70 mm) with the goal of correlating in vitro enzymatic degradation to in vivo resorption of the screw shank in the bone. As shown in Fig. 6b,d , the in vitro enzymatic degradation indicates degradation by surface erosion as compared with the control samples incubated in PBS ( Fig. 6a,c ). As shown in Fig. 6e , there was 17% mass loss after 8 weeks (56 days) of incubation. All differences between mass loss (%) of the PBS control and protease-incubated samples were considered significant for all time points using a one-tailed unpaired t -test ( P <0.05). A one-way ANOVA with Tukey’s multiple comparison test showed no significant difference ( P >0.05) in mass loss (%) for 1 and 4 week samples incubated in protease but significant differences ( P <0.05) between 1 and 8 week samples and 4 and 8 week samples. The mass loss was consistent with a second-order polynomial ( R 2 =0.999) ( Fig. 6e ). From the in vitro degradation data alone, the projected in vitro degradation to complete mass loss of the samples is ~7 months. However, this cannot be directly correlated to in vivo degradation, as more than one enzyme will play a role in the degradation in vivo and other factors such as the screw breaking down into small pieces may expose more surface area. 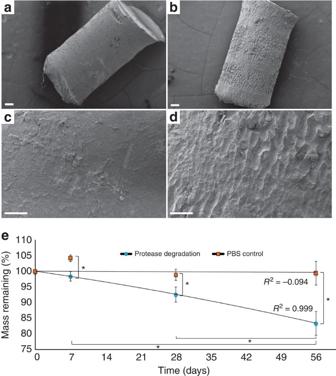Figure 6: Representative images of the enzymatic degradation. (a) Eight-week PBS control at low magnification (scale=200 μm). (b) Eight-week protease XIV at low magnification (scale=200 μm). (c) Eight-week PBS control at high magnification (scale=100 μm). (d) Eight-week protease XIV at high magnification (scale=100 μm). (e) Percent mass remaining of silk screw material as a function of time in PBS and in 5.0 U ml−1of protease XIV with curve fits and error bars (s.d.) (n=3 for each time point). A one-way ANOVA with Tukey’s multiple comparison test showed no significant difference (P>0.05) in mass loss for 1 and 4 week samples incubated in protease but significant differences (P<0.05) between 1 and 8 week samples and 4 and 8 week samples. All differences between mass loss of the PBS control and protease-incubated samples were considered significant for all time points using one-tailed unpairedt-test (P<0.05). The mass loss due to protease XIV was consistent with a second-order polynomial (y=−0.0012x2−0.229x+100.05;R2=0.999). Figure 6: Representative images of the enzymatic degradation. ( a ) Eight-week PBS control at low magnification (scale=200 μm). ( b ) Eight-week protease XIV at low magnification (scale=200 μm). ( c ) Eight-week PBS control at high magnification (scale=100 μm). ( d ) Eight-week protease XIV at high magnification (scale=100 μm). ( e ) Percent mass remaining of silk screw material as a function of time in PBS and in 5.0 U ml −1 of protease XIV with curve fits and error bars (s.d.) ( n =3 for each time point). A one-way ANOVA with Tukey’s multiple comparison test showed no significant difference ( P >0.05) in mass loss for 1 and 4 week samples incubated in protease but significant differences ( P <0.05) between 1 and 8 week samples and 4 and 8 week samples. All differences between mass loss of the PBS control and protease-incubated samples were considered significant for all time points using one-tailed unpaired t -test ( P <0.05). The mass loss due to protease XIV was consistent with a second-order polynomial ( y =−0.0012 x 2 −0.229 x +100.05; R 2 =0.999). Full size image In vivo biocompatibility of the silk screws A total of 28 screws were inserted unilaterally into the left hind limb of the rats. No screws failed during implantation and all screws were able to be inserted identically to current metallic devices where a pilot hole is drilled and the screw inserted without pre-tapping of the hole. During implantation, the screws came into contact with blood and surrounding soft tissue but still maintained their mechanical integrity for implantation. This result substantiates prior claims that the silk material does not swell quickly enough to create complications during surgery despite the presence of fluids. Immediately after surgery, after the effects of anaesthesia diminished, the rats were mobile on all four legs and were able to rear up on the leg containing the screw. While this could be attributed to the lingering effects of anaesthesia or the pain medication, the similar findings were observed when the rats were examined at 3–4 days post surgery. Throughout the 4 and 8 week periods, the rats continued to exhibit mobility on all four extremities without showing any visible signs of pain, discomfort or distress. Two animals experienced wound dehiscence but were treated with the antibiotic Baytril: the wound closed by itself and did not need further attention. Explants were isolated and characterized with photographs ( Fig. 7a ) to show that the screws did not back out of the bone and there were no visible negative reactions. 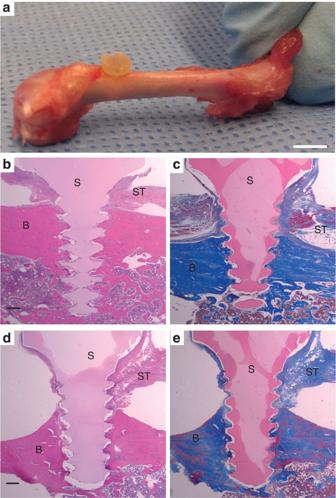Figure 7: Histological comparison of the silk screws. Analysis was performed after 4 (n=10) and 8 (n=6) weeksin vivo.(a) Silk screw and bone interface after 4 weeksin vivo. Screw did not back out and remained fixed in the femur (scale=3 mm). Cross-sections ofin vivosilk screws within bone at 4 weeks (b,c) and 8 weeks (d,e) (scale=800 μm). The screws (S) retain their position at both 4 and 8 weeks following placement, and sections show continued remodelling of adjacent bone (B), with no evidence of inflammatory reaction in bone or soft tissue (ST). Hematoxylin and eosin stains (bandd) and Masson trichrome stains (cande) at × 20 power. Figure 7: Histological comparison of the silk screws. Analysis was performed after 4 ( n =10) and 8 ( n =6) weeks in vivo. ( a ) Silk screw and bone interface after 4 weeks in vivo . Screw did not back out and remained fixed in the femur (scale=3 mm). Cross-sections of in vivo silk screws within bone at 4 weeks ( b , c ) and 8 weeks ( d , e ) (scale=800 μm). The screws (S) retain their position at both 4 and 8 weeks following placement, and sections show continued remodelling of adjacent bone (B), with no evidence of inflammatory reaction in bone or soft tissue (ST). Hematoxylin and eosin stains ( b and d ) and Masson trichrome stains ( c and e ) at × 20 power. Full size image To confirm biocompatibility and initiation of the remodelling process, the samples were prepared in paraffin blocks for histological staining with hematoxylin and eosin and Masson trichrome stains. As described previously, screws were also characterized by performing pull-out strength testing. As shown in Fig. 8 , there was recruitment of multinucleated, macrophage-like cells, possibly representing osteoclasts and early resorption of the screw at the periphery, paired with early osteoblast deposition of osteoid. Furthermore, there were multinucleated, macrophage-like cells with adjacent resorption of screw material and active osteoblasts with osteoid deposition. Although not quantifiable at this point, the early resorption of the screw material at 4 and 8 weeks in vivo is consistent with the enzymatic degradation in vitro in terms of method of degradation as both appear to degrade by surface erosion. 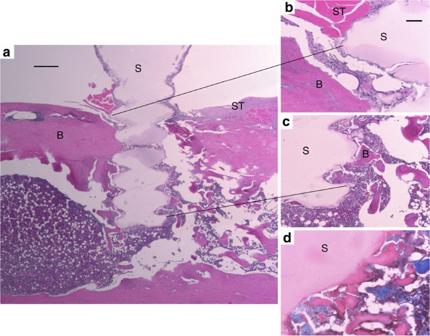Figure 8: Histological characterization of the silk screws. Analysis was performed after 4 weeksin vivo(n=10). (a) Hematoxylin and eosin stain at × 20 power: a cross-section of the screw (S) can be seen within surrounding bone (B) and soft tissue (ST) (scale=400 μm). Higher magnification (scale=60 μm) (b) demonstrates recruitment of multinucleated, macrophage-like cells, possibly representing osteoclasts for early resorption of the screw ( × 200), and (c) osteoblast deposition of osteoid to form early bone-modelling units ( × 100). Masson trichrome stain at × 400 (d) highlights the resorption of screw material and active bone formation. No significant accumulation of inflammatory cells is present. Figure 8: Histological characterization of the silk screws. Analysis was performed after 4 weeks in vivo ( n =10). ( a ) Hematoxylin and eosin stain at × 20 power: a cross-section of the screw (S) can be seen within surrounding bone (B) and soft tissue (ST) (scale=400 μm). Higher magnification (scale=60 μm) ( b ) demonstrates recruitment of multinucleated, macrophage-like cells, possibly representing osteoclasts for early resorption of the screw ( × 200), and ( c ) osteoblast deposition of osteoid to form early bone-modelling units ( × 100). Masson trichrome stain at × 400 ( d ) highlights the resorption of screw material and active bone formation. No significant accumulation of inflammatory cells is present. Full size image Figures 8a and 7b–e are representative perspective images of a silk screw in a rat femur. The conical screw head can be seen above the cortical bone and the screw threads are fixed in the bone. These images show that there are boney units in between the threads of the screw. After 4 ( Fig. 7b,c ) and 8 ( Fig. 7d,e ) weeks in vivo , it is a good sign that the screw does not simply look ‘forced’ into the pilot hole since the bone mirrors the thread profile of the screw. The screw most likely cut the threads as it is unlikely to see ingrowth of bone in the cortical area after 4 weeks. It should be noted that the tissue in histological images is often folded or pushed during sectioning. It can be stated with confidence that there are no large voids in the bone in these images but simply artefacts of histology. Conventional resorbable fixation devices provide benefits over metallic variants; however, they present laborious implantation requirements and significant limitations remain that preclude their use in broader clinical applications. Silk screws were implanted identically to current metallic fixation procedures where a pilot hole is drilled and a self-tapping screw inserted. The silk-based screws were well tolerated and initiated the typical bone-remodelling processes. After 4 and 8 week time points in vivo , there was early resorption of the silk screw. Future material iterations may involve the incorporation of bioactive compounds such as BMP-2 to promote bone ingrowth or antibiotics to prevent infection [19] , [20] , [21] , [22] , [23] , [32] , [33] . Such factors can be used to modulate healing and promote remodelling of bone. Silk plates also showed utility in implantation feasibility in vitro , as the application of water allowed malleability of the plates. Rather than having to pre-shape the plates to the exact curvature of the bone, as is the case with current resorbable devices, the plates conform to the shape of the bone and held in place after the insertion of the screws. This trait eliminates unnecessary effort by the surgeon, as the silk plates are able to actively adapt to the shape of the bone without heat treatment. Nevertheless, future studies are needed to characterize whether the hydrated silk plates maintain the required mechanical support for implantation and fixation. While swelling and hydration of the material are an obvious concern, the swelling timeline shows that there should not be a concern for losing mechanical integrity during implantation, as the material did not take up a significant amount of water or change diameter until after 8 min in vitro . Furthermore, 28 screws were inserted into rat femurs for characterization, of which none failed during implantation. With these successful outcomes with silk plates and screws, further enhancements can be envisioned in terms of mechanical properties. In some cases, the screws and plates may also need to be tuned to degrade in a shorter time frame to allow for dynamic transfer of the load back to the healing bone. Coating or incorporating the silk devices with bioactive compounds such as BMP-2 and other pharmaceuticals could provide benefits not successfully utilized in bone fixation systems at present. A limitation of the current study is the lack of a PLGA control group. Due to the manufacturing process, the silk screws had machine screw threads rather than bone screw threads and thus do not have the same geometry as PLGA screws as presented in the literature. Thus, geometrically dependent tests such as pull-out strength cannot be compared with literature values for PLGA screws. While we do not expect to see any major differences, the histological characterization of the in vivo implants may be altered as well with a different geometric profile interacting with the bone. In the present study, we demonstrated the feasibility of silk as a moudling and machinable biomaterial system for craniofacial devices. Silk has been utilized in formats for biomedical applications including sponges, fibres, foams, but not previously as a solid, hard, compact medical device. The silk material was easily machinable to different geometries and sizes allowing for flexibility in future designs. The silk screws in this study exhibited comparative shear properties to resorbable PLGA materials and were biocompatible and remained fixed in the bone up to 4 and 8 weeks. The screws were self-tapping eliminating the need for a two-step implantation process as is the case with current resorbable screws. The plates adapted to the curvature of the bone with the application of water and did not require a time-dependent heating step and pre-shaping. The versatility of silk protein will act as a benefit in future studies with future material iterations. Preparation of vacuum-dried silk Silk was prepared using our established purification protocols [34] , [35] . Taiwanese Bombyx mori cocoons were boiled for 30 min in aqueous 0.02 M Na 2 CO 3 (Sigma-Aldrich, USA) and then rinsed for 3 × 30 min in distilled water to remove the Na 2 CO 3 and sericin. The degummed cocoons were allowed to dry for more than 12 h and then subsequently dissolved in 9.3 M LiBr (Sigma-Aldrich, USA) solution at 60 °C for 3–4 h. The solution was dialysed for 2 days in distilled water using Slide-a-Lyzer dialysis cassettes (MWCO 3,500, Pierce, USA). The solution was centrifuged for 2 × 20 min at 18,000 r.p.m. The concentration was determined by measuring a volume of solution and the final dried weight. The final solution, 6–8 w/v%, was frozen for 2–5 days and vacuum dried at −20 or 0 °C until complete sublimation and stored in ambient conditions covered with tin foil to prevent any rehydration of the lyophilized solution until used in the processing steps below. The drying temperature was chosen on the basis of the speed of freeze drying, as higher temperature allowed quicker drying. Preparation of HFIP silk solutions The vacuum-dried silk was resolubilized in HFIP (Fluka Analytical, Sigma-Aldrich, USA) to generate solutions for preparation of the devices. Before dissolving in HFIP, the vacuum-dried silk was processed in a Waring blender so that the pieces could be packed into a syringe. For 25 w/v% silk in HFIP, 3 g of vacuum-dried silk was added to 30 ml syringes, then 9 ml of HFIP was added. The solubilized HFIP silk solutions were stored at ambient temperatures until used in the moudling steps below. Preparation of HFIP silk screw and plate blanks for machining Silk screw blank moulds were prepared using wax from MachinableWax.com (USA) and machined to 1.3 in (3.30 cm) height with 6 through holes of 0.30 in (0.76 cm) diameter. A thin wafer of 0.10 in (0.25 cm) was also machined to act as a base for the mould. The thin wafer was attached to the base of the mould by melting both edges of the wax and then allowing it to dry. Silk plate blank moulds were prepared using wax that was machined into a rectangular mould with inner dimensions of 1.75 × 1.75 × 1.3 in [3] (4.45 × 4.45 × 3.30 cm 3 ). Once the screw and plate moulds were filled with HFIP silk solution, they were placed in methanol (Fisher Scientific, USA) for 3–4 days to induce the β-sheet conversion and also to displace the HFIP. Subsequently, a methanol-to-water gradient was used and water was added at 4 × 1 h intervals to slowly transition the solution from 100% methanol and HFIP to 100% water. Post-gradient water changes were used to remove excess HFIP. The materials were then dried in a fume hood for at least 1 week, baked in a 60 °C oven for at least 5 days and then autoclaved prior to machining for stability. Machining of silk screws and plates The silk blanks were machined using a MicroLux True-Inch 7 × 16 Variable Speed Lathe (Micromark, USA). For the screws, the blanks were cut to the outside diameter and head diameter of the desired screw size. While the screw remained attached to the blank on the lathe, a 1–72 NF Die 13/16 OD (McMaster-Carr, USA) was used to machine the threads into the screw shank. The screw was cutoff behind the head. A diamond cutter was mounted to the lathe and a slot was cut in the screw heads. For the plates, the diamond cutter or sand paper was used to reduce the oversized blank into desirable plate thicknesses and a razor blade was used to cut the plates into various geometries. Alternatively, machine tools including a mill and band saw were used to cut the plates to the desired geometries. The silk bone screw/plate processing is depicted in Fig. 1 . Structural and morphological analysis Conformation of the silk screws were analysed with a JASCO FTIR 6200 spectrometer (Jasco, USA) using a MIRacle-attenuated total reflection accessory with Ge crystal (Pike Technologies, USA) and analysis was performed as previously described [36] . Fourier self-deconvolution of the amide I region was performed using OPUS 5.0 software (Bruker Optics, USA) with a half bandwidth of 27 cm −1 and a noise reduction factor of 0.3. For surface morphological analysis, samples were sputter coated for 90–120 s and then imaged using a ZEISS EVO MA10 SEM (Carl Zeiss, Germany). Mechanical properties The double lap shear test consisted of three consecutive stainless steel plates with an aligned 1.50 mm hole for dry shear testing and a 1.65 mm hole for hydrated shear testing. The 1.50 mm silk pins were produced to fit tightly through the fixture. The fixture was mounted into an Instron 3366 (Instron, USA) test frame. The bottom fixture remained stationary while the top fixture was compressed at a rate of 5.0 mm min −1 until fracture of the silk pin [28] . The maximum stress (MPa) was reported. Tests were performed in dry and hydrated environments by immersion in Dulbecco’s PBS (Sigma-Aldrich, USA) solution at 37 °C for greater than 72 h. The tests were then performed in a 37 °C bath of PBS. Pull-out strength consisted of an artificial bone block (Sawbones, USA) in accordance with ASTM standard F1839-08 (Standard Specification for Rigid Polyurethane Foam for Use as a Standard Material for Testing Orthopaedic Devices and Instruments) to fix the threads and a stainless steel screw head holder. The artificial bone block was drilled with a #53 drill bit (1.5 mm diameter) but was not tapped. The 1–72 machine style silk screws were generated, placed in the head holder and then screwed into the artificial bone block. The head holder was then fastened to an Instron 3366 test frame and extended in the tensile direction at a rate of 5.0 mm min −1 (ASTM standard F2502-11). Tests were performed in dry and hydrated environments by immersion in PBS solution at 37 °C for greater than 72 h. The tests were then performed in a 37 °C bath of PBS. In vitro enzymatic degradation The degradation of the silk screws was studied using protease XIV (Sigma-Aldrich, USA) with an activity of 5 U ml −1 following our published procedures [32] , [37] . Silk plugs (~0.0065, g, ~1.50 mm major diameter, ~3.00 mm overall length) were placed in well plates with 2 ml of PBS (pH 7.4) containing protease and PBS alone for control at 37 °C. The enzyme solution was replaced every 24–48 h with freshly prepared solution. Samples were killed at 1, 4 and 8 weeks, and dried, weighed and imaged using an SEM to determine degradation. In vitro swelling properties For in vitro testing, the silk material was machined, weighed to determine the dry weight of the sample (Wd) and then immersed in 37 °C PBS for various amounts of time (0 min, 1 min, 2 min, 4 min, 8 min, 15 min, 30 min, 60 min, 2 h, 4 h, 24 h, 48 h and 72 h) and observed for changes in weight and diameter to signify fluid uptake and swelling ( n =6 per time point). Surface moisture was removed from the sample by wiping with a Kimwipe (Kimberly-Clark, USA), the wet weight of the sample taken (Ws) and the major diameter was measured. The swelling ratio and water uptake (%) were calculated. In vivo swelling properties Animal studies were conducted under approved protocol #M2010-121 and amendments were approved on June 18, 2012 (#M2010-121A-1) at Tufts University. For the studies, 280 g, 20-week-old female Sprague–Dawley Rats (Charles River Laboratories International, Inc., USA) were anaesthetized with isoflurane at 4% concentration in oxygen for induction and 2.5–3% for maintenance. All samples were sterilized by autoclaving prior to implantation with a dry cycle at 25 min of steam cycle and 15 min of drying. Silk screws were implanted bilaterally, subcutaneously on the back of the rats. Rats were killed at 4 weeks ( n =12). The screws were removed, cleaned of excess tissue and weighed (Ws). The screws were then allowed to dry in excess of 2 weeks and then weighed (Wd). As described previously, the swelling ratio and water uptake (%) were calculated based on the dry weight (Wd) and wet weight (Ws). In vivo characterization and implantation technique All samples were sterilized by autoclaving prior to implantation with a dry cycle at 25 min of steam cycle and 15 min of drying. Animal studies were conducted as described in the above section, In vivo swelling properties. The incision area was shaved and disinfected with a povidone-iodine scrub. A 5–10 mm longitudinal incision was made laterally along the left hind limb. The fascia was separated between the vastus lateralis and biceps femoris and followed the length of the femur to expose the distal end. A hole with a diameter of 1.5 mm and length of 3 mm was drilled through one of the cortices with a Synthes Electric Pen Drive (Synthes, USA) and drill bit with drill stop. The screw was inserted into the femur manually with a screw driver to rotate the screw and forceps to hold the screw in the desired location. The screws were 1–72 machine screw designations with a diameter of 1.70 mm. The incision was closed using a simple interrupted pattern with 5-0 Vicryl suture and overlaid with tissue glue. Screws were inserted unilaterally to prevent complete immobilization of the animal. Buprenorphine was administered at a dosage of 0.01 mg kg −1 pre-op and pro re nata (as needed with visible signs of distress). The animals were killed at 4 ( n =10) and 8 ( n =6) weeks and assessed histologically to determine host response and signs of bone remodelling and screw resorption. There are a higher number of samples for the 4 week study due to initial pilot studies focusing on feasibility of silk screw implantation. The femur was removed and the bone sectioned ~4 mm from either side of the screw head. The samples were fixed in 10% formalin solution (Sigma-Aldrich, USA) immediately after retrieval, then sent to Beth Israel Deaconess Medical Center for histological preparation and characterization. Histological preparation The bone specimens were placed in Surgipath Decalcifier (Leica, USA) at room temperature for 8 h or until the bone became flexible. Following decalcification, tissue was processed with ethanol and xylene, and then embedded in paraffin on an automatic processor. Paraffin blocks of each specimen were then sectioned along the long axis of the bone and through the screw at 5 μ intervals. Sections were baked on glass slides at 60° C and then stained on an autostainer. Sections through the center of each specimen were stained with hematoxylin and eosin (Fisher Scientific, USA) or Masson trichrome stain. In vivo pull-out strength tests Pull-out strength tests were performed at 4 ( n =6) and 8 ( n =6) weeks. Screws were inserted identically as described above but inserted so that there was a minimum distance between the bottom of the screw head and femur of 1 mm. This was performed by placing forceps (tip width=1 mm) in between the screw head and femur to allow for proper spacing. The spacing was necessary to ensure the head could be attached to the pull-out strength testing apparatus. After the animals were killed, the femur was dislocated from the hip and the entire leg without removing any tissue was wrapped in a damp cloth and frozen at −20 °C until testing. Prior to testing, the femurs were placed in a 4 °C refrigerator for 2 days and then allowed to equilibrate to room temperature for 3 h. The femur was isolated and all soft tissues were removed. Immediately after removal of soft tissue, the femur and screw were mounted to a testing block with zip ties and mounted on the Instron 3366 testing frame as described previously. The samples were tested immediately to ensure a hydration state similar to in vivo . Statistics All experiments were run with a minimum of n =3 for each data point. Statistical analysis was performed using GraphPad Prism software. Statistical tests included one-way ANOVA with Tukey’s multiple comparison test or Dunnett’s multiple comparison test, unpaired t -test and unpaired t -test with Welch’s Correction. Differences were considered significant when P ⩽ 0.05. Regression analysis was performed using Microsoft Excel. How to cite this article: Perrone, G.S. et al. The use of silk-based devices for fracture fixation. Nat. Commun. 5:3385 doi: 10.1038/ncomms4385 (2014).